Autotransporters but not pAA are critical for rabbit colonization by Shiga toxin-producingEscherichia coliO104:H4 The outbreak of diarrhoea and haemolytic uraemic syndrome that occurred in Germany in 2011 was caused by a Shiga toxin-producing enteroaggregative Escherichia coli (EAEC) strain. The strain was classified as EAEC owing to the presence of a plasmid (pAA) that mediates a characteristic pattern of aggregative adherence on cultured cells, the defining feature of EAEC that has classically been associated with virulence. Here we describe an infant rabbit-based model of intestinal colonization and diarrhoea caused by the outbreak strain, which we use to decipher the factors that mediate the pathogen’s virulence. Shiga toxin is the key factor required for diarrhoea. Unexpectedly, we observe that pAA is dispensable for intestinal colonization and development of intestinal pathology. Instead, chromosome-encoded autotransporters are critical for robust colonization and diarrhoeal disease in this model. Our findings suggest that conventional wisdom linking aggregative adherence to EAEC intestinal colonization is false for at least a subset of strains. Diarrhoeagenic Escherichia coli is classified into six different ‘pathotypes’ primarily based on the patterns and mechanisms by which these pathogens adhere to cultured human cells and on presumed mechanisms of virulence (for example, toxin production) [1] . Enteroaggregative E. coli (EAEC) are distinguished by their characteristic aggregative ‘stacked brick’ pattern of adherence to HEp-2 cells, a phenotype that is mediated by aggregative adherence plasmid (pAA)-encoded fimbriae [2] . EAEC is increasingly associated with acute and persistent diarrhoeal disease in a variety of endemic settings in both the developed and developing world and in travellers [3] , [4] . Furthermore, EAEC has been known to cause large outbreaks of diarrhoea [2] . Notably, in 2011, there was a large food-borne outbreak of diarrhoea and haemolytic uraemic syndrome (HUS) centred in Germany [5] caused by an atypical EAEC strain that produced Shiga toxin (Stx) [6] , [7] . This serogroup O104:H4 strain was classified as EAEC because of the presence of a pAA and the associated aggregative adherence on cultured cells [8] . Most EAEC strains do not produce Stx, a potent inhibitor of protein synthesis that can cause HUS and is more typically a defining feature of enterohaemorrhagic E. coli (EHEC) [9] . Understanding of the factors and mechanisms that enable EAEC to colonize the intestine and cause diarrhoea has been hampered by the marked genetic heterogeneity of EAEC strains, both at chromosomal and pAA-encoded loci [1] , [2] . A variety of putative virulence factors, including plasmid- and chromosome-encoded toxins and fimbriae, have been described, but to date no single or set of putative virulence-associated gene(s) is found in all EAEC [1] . Studies of EAEC pathogenicity have also been hindered by a lack of suitable animal models for testing the importance of putative colonization and virulence factors [1] . Some initial studies were plagued by a lack of reliable intestinal colonization [10] , [11] , [12] , perhaps due to the presence of normal intestinal flora. Although treatment of animals with antibiotics can prevent this difficulty, colonized animals often do not exhibit intestinal manifestations of disease, such as diarrhoea and inflammation, either in response to classical (Stx − ) EAEC or in response to the outbreak-linked Stx2 + isolates [12] , [13] , [14] . For example, although outbreak-linked O104:H4 isolates induce kidney damage in ampicillin-treated mice [14] , they do not cause pathological changes in the murine intestine. In addition, studies with antibiotic-treated animals have not reliably confirmed the importance of factors known to be important for pathogenesis in humans, such as the type 3 secretion system that is critical for the virulence of EHEC [15] , [16] . In contrast, our previous studies using infant rabbit models of EHEC, Vibrio cholerae and V. parahaemolyticus infection have revealed close similarities between factors required in humans and infant rabbits for intestinal colonization, induction of diarrhoea and histopathological signs of disease, suggesting that rabbits are excellent model hosts for the investigation of enteric pathogens [17] , [18] , [19] , [20] . Here we report the development of an infant rabbit-based animal model of intestinal disease caused by Stx-producing E. coli O104:H4, which we use to decipher the factors that enable this pathogen to colonize the intestine and cause disease. As anticipated, our studies confirm the causal role of Stx in diarrhoea. In addition, they suggest that putative adherence fimbriae and other pAA-encoded factors are not required for intestinal colonization by EAEC, and that chromosome-encoded autotransporters are more significant for robust colonization and subsequent induction of diarrhoeal disease. Stx + EAEC induces intestinal disease in infant rabbits To investigate the pathogenicity of E. coli O104:H4, 2-day-old rabbits were orogastrically inoculated with a clinical isolate from the 2011 German outbreak, C227-11 (here referred to as C227), whose genome had been sequenced [6] . 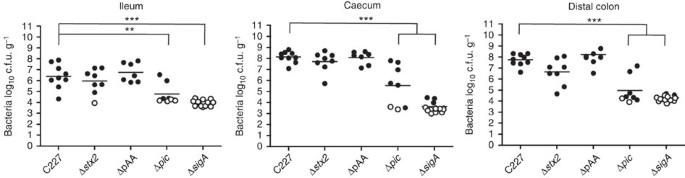Figure 1: Intestinal colonization in infant rabbits inoculated withE. coliC227 or isogenic mutants. Concentration (c.f.u. g−1) of bacteria recovered 3 days PI from homogenates of intestinal tissues from rabbits infected with the indicated strain. Data points represent individual rabbits (C227,n=9; Δstx2,n=8; ΔpAA,n=7; Δpic,n=8; ΔsigA,n=13). Open symbols represent the limit of detection for samples from which no c.f.u. were isolated. Bars show the geometric mean. Statistical analysis was performed using one-way analysis of variance and Bonferroni’s multiple comparison post-test; **P<0.01 and ***P<0.001. Nearly all rabbits inoculated with C227 developed diarrhoea and/or intestinal fluid accumulation by 3 days post inoculation (PI), while mock-infected rabbits did not display any signs of disease ( Table 1 ). The majority of C227 colony-forming units (c.f.u.) were detected in homogenates of the caecum and colon of infected animals, although bacteria were also recovered from the distal small intestine ( Fig. 1 ). Peak colonization occurred 2–3 days PI and diminished thereafter ( Fig. 2 ). Immunofluorescence microscopy revealed that C227 cells were primarily present as large aggregates in the intestinal lumen, and were often apparently attached to luminal contents ( Fig. 3a and Supplementary Fig. 1 ). Individual C227 cells were also attached to the epithelial surface but did not markedly disrupt the underlying epithelium. Statistically significant increases in inflammation (marked by infiltration of heterophils (rabbit equivalent of neutrophils)) and apoptosis of epithelial cells were evident in the colonic and caecal epithelia but not in the small intestines of infected rabbits ( Fig. 3b,c and Supplementary Fig. 2 ). Breaching of the colonic epithelial permeability barrier, measured as increased uptake of biotin relative to mock-infected animals, was also observed ( Fig. 3d ), but renal pathology was not detected. Our data suggest that diarrhoea in response to C227 infection is not linked to marked disruption of the intestinal epithelium, as seen with some pathogens [20] , but instead is associated with inflammation and more subtle alterations in epithelial barrier function. Table 1 Diarrhoea in infant rabbits inoculated with the indicated strains. Full size table Figure 1: Intestinal colonization in infant rabbits inoculated with E. coli C227 or isogenic mutants. Concentration (c.f.u. g −1 ) of bacteria recovered 3 days PI from homogenates of intestinal tissues from rabbits infected with the indicated strain. Data points represent individual rabbits (C227, n =9; Δ stx2 , n =8; ΔpAA, n =7; Δ pic , n =8; Δ sigA , n =13). Open symbols represent the limit of detection for samples from which no c.f.u. were isolated. Bars show the geometric mean. Statistical analysis was performed using one-way analysis of variance and Bonferroni’s multiple comparison post-test; ** P <0.01 and *** P <0.001. 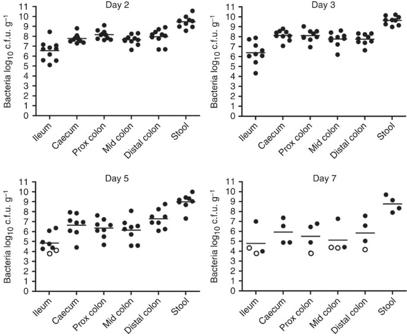Figure 2: Kinetics of C227 colonization in infant rabbits. Concentration (c.f.u. g−1) of bacteria recovered from homogenates of intestinal tissues or stools from rabbits infected with wt C227 at different times after infection. Data points represent individual rabbits (day 2,n=10; day 3,n=9; day 5,n=8; day 7,n=4). Open symbols represent the limit of detection for samples from which no c.f.u. were isolated. Bars show the geometric mean. Full size image Figure 2: Kinetics of C227 colonization in infant rabbits. Concentration (c.f.u. g −1 ) of bacteria recovered from homogenates of intestinal tissues or stools from rabbits infected with wt C227 at different times after infection. Data points represent individual rabbits (day 2, n =10; day 3, n =9; day 5, n =8; day 7, n =4). Open symbols represent the limit of detection for samples from which no c.f.u. were isolated. Bars show the geometric mean. 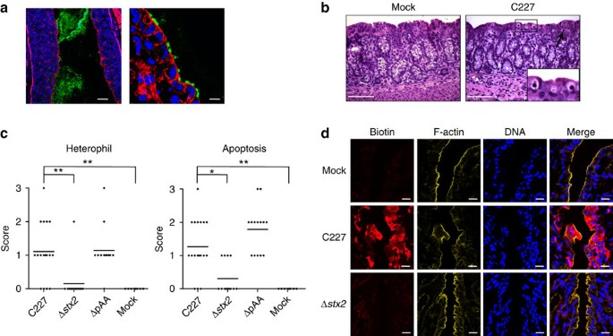Figure 3: Histopathology in infant rabbits inoculated withE. coliC227 or isogenic mutants. (a) Representative confocal micrographs showing C227 in the intestinal lumen and attached to intestinal tissue at day 3 PI in the distal colon. C227 was stained with polyclonal antisera against C227 (green) and luminal epithelial cells were counterstained with phalloidin-Alexa 568 (red) and 4',6-diamidino-2-phenylindole (DAPI; blue) to detect F-actin and nuclei, respectively. Scale bar, 100 μm (left panel) and 10 μm (right panel). (b) Representative haematoxylin and eosin-stained colonic sections from C227 and mock-infected rabbits 3 days PI showing infiltration of heterophils (arrow) and apoptosis (enlarged box). Scale bar, 100 μm. (c) Pathology scores for infiltration of heterophils and apoptosis in the distal colon of rabbits inoculated with the indicated strain. Data points represent individual rabbits from 2 and 3 days PI (C227,n=19; Δstx2,n=13; ΔpAA,n=14; Mock,n=8). Statistical analysis was performed using the Kruskal–Wallis statistic with Dunn’s post-test for multiple comparisons. *P<0.05, **P<0.01. (d) Colonic tissue from rabbits infected with the indicated strain stained with biotin (red) before sectioning, and then counterstained with DAPI (blue) and phalloidin-Alexa 633 (yellow). Scale bar, 20 μm. Full size image Figure 3: Histopathology in infant rabbits inoculated with E. coli C227 or isogenic mutants. ( a ) Representative confocal micrographs showing C227 in the intestinal lumen and attached to intestinal tissue at day 3 PI in the distal colon. C227 was stained with polyclonal antisera against C227 (green) and luminal epithelial cells were counterstained with phalloidin-Alexa 568 (red) and 4',6-diamidino-2-phenylindole (DAPI; blue) to detect F-actin and nuclei, respectively. Scale bar, 100 μm (left panel) and 10 μm (right panel). ( b ) Representative haematoxylin and eosin-stained colonic sections from C227 and mock-infected rabbits 3 days PI showing infiltration of heterophils (arrow) and apoptosis (enlarged box). Scale bar, 100 μm. ( c ) Pathology scores for infiltration of heterophils and apoptosis in the distal colon of rabbits inoculated with the indicated strain. Data points represent individual rabbits from 2 and 3 days PI (C227, n =19; Δ stx2 , n =13; ΔpAA, n =14; Mock, n =8). Statistical analysis was performed using the Kruskal–Wallis statistic with Dunn’s post-test for multiple comparisons. * P <0.05, ** P <0.01. ( d ) Colonic tissue from rabbits infected with the indicated strain stained with biotin (red) before sectioning, and then counterstained with DAPI (blue) and phalloidin-Alexa 633 (yellow). Scale bar, 20 μm. Full size image Stx is essential for C227-induced diarrhoea and histopathology C227, like other isolates from the 2011 German outbreak, encodes numerous putative virulence factors, including the prophage-borne stx 2 AB, which encode the A and B subunits of Stx2. This toxin, a potent inhibitor of protein synthesis, is a critical virulence factor in EHEC both in infected humans and in our infant rabbit model of EHEC infection [9] , [17] . C227 and EHEC O157:H7 produce similar amounts of Stx2 in vitro ( Supplementary Fig. 3 ). Notably, a C227 mutant lacking stx 2 AB (Δ stx2 ) colonized the rabbit intestine in a similar manner as the wild–type (wt) strain; however, animals inoculated with this mutant did not exhibit diarrhoea or impairment of the colonic epithelial permeability barrier, and they showed a marked reduction in heterophil infiltration and apoptosis in the colonic and caecal epithelium relative to C227-infected animals ( Table 1 , Figs 1 and 3c,d ). Collectively, these observations are consistent with previous observations linking Stx2 to diarrhoea and inflammation in rabbits infected with EHEC [17] and to apoptosis in toxin-treated animals [21] . They also suggest that Stx2 disrupts the intestinal permeability barrier in C227-infected animals, potentially either directly, by intoxicating epithelial cells, or indirectly, through induction of inflammation and apoptosis. The critical role of Stx2 in rabbit pathogenesis supports the prevailing analysis during the German outbreak that the presence of a prophage encoding stx 2 AB rendered outbreak-linked strains far more pathogenic than typical EAEC isolates [6] , [22] . This finding is also compatible with results from a study of antibiotic-treated mice infected with E. coli O104:H4 +/− a toxin-encoding prophage [14] ; however, our study more conclusively links virulence to the presence of Stx2, as it rules out possible effects of other phage-encoded factors, such as a restriction/modification system previously shown to modulate expression of numerous bacterial loci [23] . pAA is dispensable for colonization by O104:H4 strains Although highly heterogeneous in gene content, EAEC strains harbour a plasmid (pAA) that mediates aggregative adherence to tissue-cultured cells (via plasmid-encoded aggregative adherence fimbria) and encodes several additional putative virulence factors [24] . We isolated a C227 derivative that had spontaneously lost its pAA, which as expected no longer exhibited aggregative adherence to cultured HEp-2 cells ( Fig. 4a ). Surprisingly, the overall accumulation and intestinal distribution of the plasmid-free strain in rabbit intestines were equivalent to those of the wt strain ( Fig. 1 and Supplementary Fig. 4 ), and the two strains induced equivalent frequency/intensity of diarrhoea, inflammation and apoptosis ( Fig. 3c and Table 1 ). In addition, comparative analyses of C227 gene expression under laboratory conditions (in Luria-Bertani (LB) medium) and during infection (assessed using RNA isolated from organisms within the caecal fluid of infected rabbits) revealed that of the 51 pAA genes that were differentially expressed between these two conditions, 42 (82%) showed reduced expression in vivo ( Fig. 4b ). These 42 genes included several putative virulence genes, for example, the putative virulence regulator aggR , aggACD (encodes AAF-I), aap (dispersin) and aatPABCD (the dispersin translocator) ( Fig. 4b , Supplementary Table 1 ). Thus, our analyses suggest that despite their impact on bacterial adhesion in vitro , pAA-encoded adhesins and other gene products are not required for intestinal colonization or subsequent development of C227-based intestinal pathology in this animal model of disease. 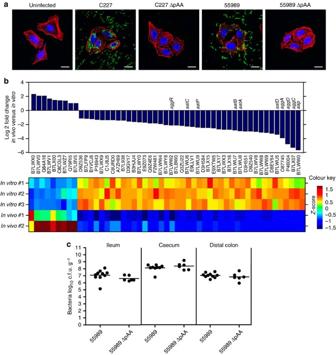Figure 4: The role of pAA in virulence of O104:H4 EAEC. (a) Adherence of EAEC to HEp-2 cells. HEp-2 cells infected with the indicated strain were stained with polyclonal antisera against C227 (green) and counterstained with phalloidin-Alexa 568 (red) and DAPI (blue) to detect F-actin and nuclei, respectively. Scale bar, 20 μm. (b) Relative expression of pAA genes that are differentially expressedin vivo(rabbit caecal fluid) versusin vitro(LB) at a false discovery rate<0.01. Graphic and heat map representation of the 51 genes that are differentially expressed in two replicates of C227in vivorelative to three replicatesin vitro. TheZ-score reflects the degree of decreased (Z-score<0) or increased (Z-score>0) abundance, computed by subtracting the mean of the log-transformed expression values and dividing by the s.d. for each gene over all samples scored. (c) Concentration (c.f.u. g−1) of bacteria recovered 2 or 3 days PI from intestinal homogenates of tissues from rabbits infected with the indicated strain. Data points represent individual rabbits (55989,n=10; 55989 ΔpAA,n=6). Bars show the geometric mean. Figure 4: The role of pAA in virulence of O104:H4 EAEC. ( a ) Adherence of EAEC to HEp-2 cells. HEp-2 cells infected with the indicated strain were stained with polyclonal antisera against C227 (green) and counterstained with phalloidin-Alexa 568 (red) and DAPI (blue) to detect F-actin and nuclei, respectively. Scale bar, 20 μm. ( b ) Relative expression of pAA genes that are differentially expressed in vivo (rabbit caecal fluid) versus in vitro (LB) at a false discovery rate<0.01. Graphic and heat map representation of the 51 genes that are differentially expressed in two replicates of C227 in vivo relative to three replicates in vitro . The Z -score reflects the degree of decreased ( Z -score<0) or increased ( Z -score>0) abundance, computed by subtracting the mean of the log-transformed expression values and dividing by the s.d. for each gene over all samples scored. ( c ) Concentration (c.f.u. g −1 ) of bacteria recovered 2 or 3 days PI from intestinal homogenates of tissues from rabbits infected with the indicated strain. Data points represent individual rabbits (55989, n =10; 55989 ΔpAA, n =6). Bars show the geometric mean. Full size image To investigate whether pAA plays a more significant role in intestinal colonization by other O104:H4 strains, we isolated a derivative of 55989 (a non-Stx-producing EAEC O104:H4 strain [25] ) that lacked its AA plasmid. As anticipated, loss of pAA eliminated 55989’s aggregative adherence to HEp-2 cells ( Fig. 4a ). However, there was no difference between intestinal colonization by 55989 harbouring or lacking pAA ( Fig. 4c ). Thus, our experiments suggest that at least for serogroup O104:H4 strains, AA plasmids do not play a significant role in intestinal adhesion or colonization. Our results are consistent with a very recent analysis of bacterial isolates from the German outbreak and a recent study using ampicillin-treated mice, in which loss of pAA during the progression of an infection was frequently detected [14] , [26] , and provide the first indication that establishment (rather than maintenance) of an intestinal infection is not necessarily dependent on pAA. However, we should note that analyses of human isolates did suggest that the presence of pAA augments the likelihood of HUS associated with Stx2 + EAEC infection. This hypothesis cannot be evaluated using our animal model, since infant rabbits do not develop HUS or other renal pathology, either in response to EHEC infection or to Stx2 + EAEC. Thus, while our data suggest that pAA does not contribute to establishment of intestinal infections by C227 or other O104:H4 EAEC, which is a prerequisite for induction of diarrhoea and intestinal pathology, we cannot fully rule out a role for the plasmid in subsequent stages of E. coli O104:H4-induced disease or exclude the possibility that distinct factors mediate disease in humans and infected animals. Whether AA plasmids promote colonization by other diverse EAEC serogroups remains an open question. SPATEs promote C227 intestinal colonization and disease Although the presence of pAA is the defining feature of EAEC, and pAA has been presumed to contribute to EAEC virulence, human volunteer studies have demonstrated that the presence of pAA is not sufficient for pathogenicity [27] . Other factors hypothesized to play a role in pathogenesis are the serine protease autotransporters of Enterobacteriaceae (SPATEs), which are produced by a variety of pathogenic E. coli , Shigella and Salmonella [28] , [29] . These autotransporter proteins are comprised of an amino-terminal signal peptide for targeting the protein to the periplasm, followed by a secreted ‘passenger’ domain (containing the serine protease) and a β domain that promotes the translocation and targeting of the passenger domain to the outer membrane in a multistep process catalysed by the Bam complex [30] , [31] . The N terminus is subsequently released from the cell via SPATE autocleavage [29] ( Fig. 5a,b ), and typically is among its producer’s most abundant secreted proteins. Almost all (95%) EAEC isolates encode at least one SPATE, while a far lower percentage of other E. coli pathotypes produce these proteins [32] . The Stx-producing EAEC O104:H4 strain that caused the German outbreak contains genes encoding three different SPATES. Two of these, sigA (refs 33 , 34 ) and pic (refs 12 , 35 ), which is encoded in two identical copies, are located on chromosomal pathogenicity islands, while the third, sepA (ref. 36 ), is found on pAA. All three SPATEs were detected in supernatants from C227 cultures as active serine proteases using an activity-based probe ( Fig. 5c ). SepA is clearly not required for C227 pathogenicity, since colonization and virulence of C227 and C227ΔpAA were indistinguishable. In contrast, deletion of either sigA or both copies of pic (which was confirmed using the activity-based assay of secreted proteins; Fig. 5c ) reduced intestinal colonization 3 days PI by ~3 orders of magnitude ( Fig. 1 ). The attenuation in the colonization of the SPATE mutants was less dramatic 2 days PI ( Supplementary Fig. 4 ), suggesting that these autotransporters may promote the persistence of the pathogen in the gastrointestinal tract. As expected, the absence of these SPATEs did not alter aggregative adherence of C227 ( Supplementary Fig. 5 ). 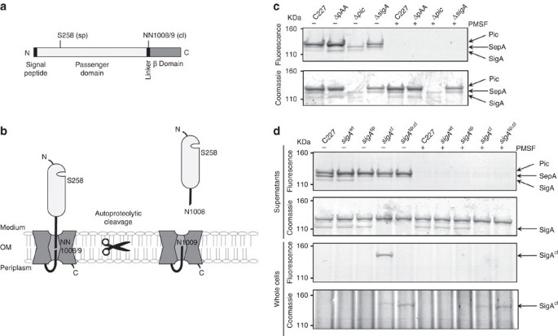Figure 5: Activity of SPATEs from C227 and isogenic mutants. (a) Domain structure and predicted catalytic serine (sp) and autocleavage sites (cl) in SigA. (b) Schematic of SigA topology and processing. (c) Activity-Based Protein Profiling (ABPP) of secreted SPATEs from C227. Supernatants from overnight cultures of the indicated strains were reacted with a serine hydrolase activity-based probe (TAMRA-FP), run on SDS–polyacrylamide gels and scanned to detect fluorescence or stained with coomassie to visualize total protein. Control samples were incubated with phenylmethylsulphonyl fluoride (PMSF), which specifically abolishes serine protease activity, before addition of TAMRA-FP. (d) ABPP of C227, its ΔsigAderivative complemented withsigAwtor the indicatedsigApoint mutants. Whole cells or supernatants from overnight cultures were assayed as inc. Full fluorescence-scanned blots and coomassie-stained gels are shown inSupplementary Fig. 8. Figure 5: Activity of SPATEs from C227 and isogenic mutants. ( a ) Domain structure and predicted catalytic serine (sp) and autocleavage sites (cl) in SigA. ( b ) Schematic of SigA topology and processing. ( c ) Activity-Based Protein Profiling (ABPP) of secreted SPATEs from C227. Supernatants from overnight cultures of the indicated strains were reacted with a serine hydrolase activity-based probe (TAMRA-FP), run on SDS–polyacrylamide gels and scanned to detect fluorescence or stained with coomassie to visualize total protein. Control samples were incubated with phenylmethylsulphonyl fluoride (PMSF), which specifically abolishes serine protease activity, before addition of TAMRA-FP. ( d ) ABPP of C227, its Δ sigA derivative complemented with sigA wt or the indicated sigA point mutants. Whole cells or supernatants from overnight cultures were assayed as in c . Full fluorescence-scanned blots and coomassie-stained gels are shown in Supplementary Fig. 8 . Full size image SigA release but not protease activity mediates colonization Analysis of a wt revertant derived from C227Δ sigA (SigA wt ) confirmed that the attenuation of C227Δ sigA results from absence of SigA: C227 SigA wt caused diarrhoea and colonized rabbit intestines in a similar manner as wt C227 ( Figs 5d and 6, Table 2 ). Unexpectedly, a sigA point mutant that lacks serine protease activity (SigA sp ; SigA S258A; Fig. 5d ) also displayed virulence equivalent to that of the wt strain ( Fig. 6 and Table 2 ), suggesting that SigA substrate cleavage does not contribute to C227 pathogenesis. However, a sigA point mutant that lacks an autocleavage site and hence is not released from the cell surface into supernatants (SigA cl ; SigA N1008A, N1009A; Fig. 5d ) was as highly attenuated in infant rabbits as C227Δ sigA ( Fig. 6 and Table 2 ). Secreted colonization factors are rare but have been described in other bacterial pathogens [37] . SigA’s precise role remains to be defined; analysis of the effects of SigA, Pic and additional SPATEs on the virulence of diverse EAEC isolates are also warranted to clarify whether this family of proteins routinely contributes to pathogenesis. Table 2 Diarrhoea in infant rabbits inoculated with C227 or isogenic sigA point mutants . 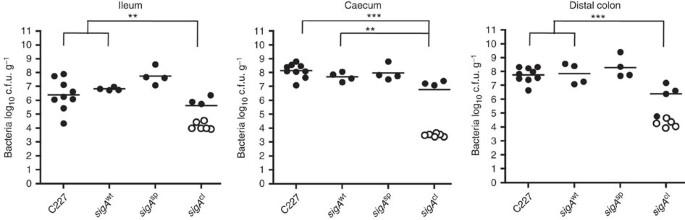Figure 6: Intestinal colonization in infant rabbits inoculated with C227 or isogenicsigApoint mutants. Concentration (c.f.u. g−1) of bacteria recovered 3 days PI from intestinal homogenates of tissues from rabbits infected with the indicated strain. Data points represent individual rabbits (C227,n=9;sigAwt,n=4;sigAsp,n=4;sigAcl,n=9). Open symbols represent the limit of detection for samples from which no c.f.u. were isolated. Bars show the geometric mean. Statistical analysis was performed using one-way analysis of variance and Bonferroni’s multiple comparison post-test; **P<0.01 and ***P<0.001. Full size table Figure 6: Intestinal colonization in infant rabbits inoculated with C227 or isogenic sigA point mutants. Concentration (c.f.u. g −1 ) of bacteria recovered 3 days PI from intestinal homogenates of tissues from rabbits infected with the indicated strain. Data points represent individual rabbits (C227, n =9; sigA wt , n =4; sigA sp , n =4; sigA cl , n =9). Open symbols represent the limit of detection for samples from which no c.f.u. were isolated. Bars show the geometric mean. Statistical analysis was performed using one-way analysis of variance and Bonferroni’s multiple comparison post-test; ** P <0.01 and *** P <0.001. Full size image Classification of diarrhoeagenic E. coli based on patterns of adherence to tissue-cultured cells [1] , [38] has been a useful heuristic, as in many cases in vitro -based classifications reflect consistent pathology in vivo . However, our findings in the infant rabbit model that pAA-based aggregative behaviour is not linked with intestinal colonization by strains classified as EAEC, coupled with the known genetic heterogeneity of EAEC isolates, suggest that at least for this subset of pathogenic E. coli , shared adherence phenotypes may have masked recognition of important colonization and virulence mechanisms. Our data further suggest that strain-specific factors and mechanisms, such as autotransporters, may play a more prominent role in pathogenicity than previously recognized. Our new infant rabbit model of EAEC infection should be extremely useful for preliminary identification and analyses of such factors. Ethics statement The animal protocols used for the studies described here were reviewed and approved by the Harvard Medical Area Standing Committee on Animals (Institutional Animal Care and Use Committee protocol number 04308, Animal Welfare Assurance of Compliance number A3431-01). All animal studies were carried out in accordance with the recommendations in the Guide for the Care and Use of Laboratory Animals of the National Institutes of Health (8th edition) and the Animal Welfare Act of the United States Department of Agriculture. Bacterial strains and plasmids and growth conditions Strains, plasmids and primers used in this study are listed in Supplementary Tables 2, 3 and 4 , respectively. The E. coli O104:H4 German outbreak strain isolate C227-11 (C227) [6] and EAEC O104:H4 strain 55989 (55989) [25] were the wt strains used in this study. Isogenic mutants of C227 were constructed by standard allele exchange techniques [39] using derivatives of suicide vectors pDS132 or pDM4 harbouring DNA regions flanking stx 2 AB , sigA and pic ( Supplementary Tables 3 and 4 ); the two identical pic copies were deleted in a sequential manner. C227Δ sigA was used as the starting strain to generate sigA wt , sigA sp , sigA cl and sigA sp,cl mutants with allele replacement vectors pDM4-flk-sigA(wt), pDM4-flk-sigA(S258A), pDM4-flk-sigA(N1008A, N1009A) and pDM4-flk-sigA(S258A, N1008A, N1009A), respectively. E. coli strain MFD pir was used as a donor strain to deliver allele exchange vectors by conjugation to recipient EAEC strains. PCR and sequencing was used to confirm all the mutants used in this study. Serial passages in culture were used to isolate C227 and 55989 mutants that lost their respective pAA plasmids, which was established by PCR tests of internal fragments for plasmid loci aggR , aatA, aatB , sepA , aap and chromosomal-encoded lacZ as a positive control ( Supplementary Fig. 6 and Supplementary Table 4 ). All strains were routinely grown in LB medium or on LB agar plates containing the appropriate antibiotics at the following concentrations: 20 μg ml −1 chloramphenicol and 200 μg ml −1 streptomycin. Growth curves of wt strains and their derivatives ( Supplementary Fig. 7 ) did not reveal detectable differences in the generation times of the strains used in this work. Infant rabbit infection studies Litters of 2-day-old New Zealand White infant rabbits (both genders) with the lactating doe were acquired from a commercial breeder. The same day, the rabbits were administered ranitidine intraperitoneally (2 μg g −1 ) and 3 h later they were orogastrically inoculated with 1 × 10 9 c.f.u. of the EAEC strain (suspended in sodium bicarbonate solution (pH 9)) using a size 4 French catheter. Following inoculation, the infant rabbits were monitored at least 2 × per day for signs of illness. At euthanasia, disease was scored as follows: no gross disease (no adherent fecal material on fur and intestines appear normal), intestinal fluid (no adherent fecal material on fur but intestines swollen with fluid), diarrhoea (liquid fecal material stains adherent to fur, and intestines swollen with fluid). The number of C227 or 55989 c.f.u. in tissue samples taken from the ileum, caecum, proximal colon, mid colon, distal colon and stools were determined after homogenization, serial dilution and plating on LB media containing 200 μg ml −1 streptomycin [19] . For sections where no colonies were detected at the lowest dilution plated, the c.f.u. were calculated using the lower limit of detection as a value. Histopathology and immunofluorescence microscopy For histological analyses, tissue sections were fixed in 10% neutral-buffered formalin, processed for paraffin embedding and stained with haematoxylin and eosin. Slides were examined using a Zeiss AxioImager M1 microscope at × 40 magnification with an AxioCamMR Camera and processed using Axio Vision 4.8 LE software (Zeiss). The slides were semiquantitatively assessed for apoptosis and infiltration of heterophils by a pathologist blinded to the origin of the tissue. Each histological parameter was evaluated on a 0–3 scale as follows: 0 (normal), 1 (mild), 2 (moderate) and 3 (severe). Tissue sections used for immunofluorescence studies were fixed in 4% paraformaldehyde (in PBS) on ice for 2 h before being placed in 30% sucrose (in PBS) at 4 °C overnight. The next day, the tissue segments were briefly washed in PBS, the outer surface was dried on filter paper and trimmed pieces were placed in optimal cutting temperature compound (Electron Microscopy Sciences, PA). Each tissue block was quick frozen over a mixture of dry ice and ethanol and stored at −80 °C before sectioning. Sections that were ~ 5 μm thick were cut, placed on glass slides and processed for immunofluorescence. Initially, optimal cutting temperature compound was removed from the tissue section by washing the slides three times in PBS (5 min each). For detection of C227, chicken polyclonal antisera generated against heat-killed C227 (Lampire) was employed in combination with an anti-IgY chicken-fluorescein isothiocyanate conjugate (Abcam). Slides were examined for fluorescence using a Zeiss LSM510 Meta upright confocal microscope at × 63 magnification. Biotin permeability Biotin was used as a tracer molecule to determine the integrity of the epithelial barrier [20] . Briefly, immediately after removal of the entire intestinal tract from mock, C227 or Δ stx2 -infected rabbits, the colonic tissue was separated while maintaining the correct orientation (that is, proximal versus distal ends). EZ-Link Sulfo-NHS-Biotin (Thermo Scientific, IL) was injected slowly (1–2 min) into the lumen via the open (cut) end of the most distal part of the colon. After 3 min, the tissue section just proximal to the site of injection was removed, fixed in 4% paraformaldehyde and processed for immunofluorescence staining as described above. Tissue sections were incubated with streptavidin linked to Alexa 546 (1/500) (S11225; Invitrogen) for 1 h at room temperature (RT) before being counterstained with phalloidin-Alexa fluor 633 and DAPI. Colonic tissue from mock, C227 or Δ stx2 -infected rabbits that were not treated with biotin exhibited no background staining following incubation with streptavidin only. HEp-2 cell adherence assay HEp-2 cell adherence assays were carried out as described previously [40] with the following modifications. HEp-2 cells (ATCC CCL-23) were grown for 24 h to 50–60% confluence on 13 mm diameter coverslips in 24-well tissue culture plates in MEM supplemented with 10% fetal calf serum (fetal bovine serum; Sigma) at 37 °C in a 5% CO 2 atmosphere. On the day of the assay, the HEp-2 cells were washed with MEM containing 1% D -mannose (Sigma-Aldrich) in PBS and 1 ml of this medium was added to each well. Infections were performed in triplicate with 25 μl per well of the indicated strain grown statically at 37 °C for 16–18 h. After 3 h of incubation at 37 °C in a 5% CO 2 atmosphere, unbound bacteria were removed by washing three times with Dulbecco’s PBS (Sigma). Cells were fixed with 3% paraformaldehyde for 20 min at RT before washing in PBS. For immunostaining, the fixed cells were quenched for 20 min with PBS/50 mM NH 4 Cl, permeabilized for 4 min in PBS/0.1% Triton X-100 and washed three times in PBS. The coverslips were then blocked for 10 min with 1% BSA in PBS, incubated with C227 chicken polyclonal antisera (1/200) 1 h at RT, washed in PBS, blocked and incubated with goat anti-chicken fluorescein isothiocyanate secondary antibody (1/200), Alexa Fluor Phalloidin 568 (1/100) and DAPI (1 μg ml −1 ) 1 h at RT in the dark. After washing three times with PBS and three times with MiliQ water, coverslips were mounted on slides using ProLong Gold anti-fade reagent (Invitrogen). RNA sequencing and analysis RNA was isolated from triplicate mid-exponential phase (O.D.≈0.6) C227 cultures grown in LB at 37 °C and from the caecal fluid of two C227-infected rabbits [41] . RNA samples were treated with RiboZero bacterial Gram-negative ribosomal removal kit (Epicentre; MRZGN126). For complementary DNA library preparation [23] , [41] , ribosomal RNA-depleted RNA was chemically fragmented and then reverse transcribed with SuperScript III (Invitrogen) using random hexamers. The cDNA was converted to double-stranded DNA, end repaired, 5′-adenylated and then ligated to DNA adapters enabling Illumina sequencing using the NEB Next mRNA-seq kit (New England BioLabs; E6100S). PCR for 16 cycles using KAPA HiFi HotStart DNA Polymerase was performed to incorporate Illumina-specific sequences and molecular barcodes. The Illumina HiSeq 2000 with a read length of 100 nucleotides was used for sequencing. Reads were mapped to the TY-2482 reference genome. A gene was included for differential expression analysis if it had more than one count per million reads in at least two samples. For the differential expression results depicted in Fig. 4b , the program edgeR was used to detect significantly differentially expressed genes at a false discovery rate<0.01. To display the expression data in Fig. 4b , expression values were converted into a z -score by subtracting the mean expression value and dividing by the s.d. for each gene over all samples scored. Gene expression data have been deposited in the Sequence Read Archive database ( www.ncbi.nlm.nih.gov/Traces/sra/ ) under accession number SRS505092 . Activity-based protein profiling (ABPP) assays To test the serine protease activity of SPATEs, 5 ml cultures were grown at 37 °C with shaking for 24 h. Filtered concentrated culture supernatants were quantified and normalized to the total protein. To analyse SPATE activity in whole cells, 200 μl of each culture were pelleted, washed with PBS and resuspended in PBS. Duplicates of 44 μl of each supernatant and whole-cell sample were prepared and phenylmethylsulphonyl fluoride (25 mM final concentration) was added to one sample to specifically inactivate serine proteases while the same amount of ethanol was added to the other sample. After incubation at 37 °C for 30 min, all samples were reacted with 2 mM of ActivX TAMRA-FP (Thermo Scientific), a serine hydrolase probe, for 1 h at RT in the dark. Samples were prepared under denaturing (1% SDS, 95 °C, 5 min) conditions and 15 μl of each sample were separated on SDS polyacrylamide 3–8% Tris-acetate gels, using standard methods [42] . Gels were fluorescence scanned using an FLA-5100 Imager Reader (Fujifilm). The protein content in the samples was visualized after separation on SDS polyacrylamide 3–8% Tris-acetate gels with coomassie [42] . Full fluorescence-scanned blots and coomassie-stained gels are shown in Supplementary Fig. 8 . Accession codes: Gene expression data have been deposited in the Sequence Read Archive database under the accession code SRS505092 . How to cite this article: Munera, D. et al . Autotransporters but not pAA are critical for rabbit colonization by Shiga toxin-producing Escherichia coli O104:H4. Nat. Commun. 5:3080 doi: 10.1038/ncomms4080 (2014).